Drying of Indian subcontinent by rapid Indian Ocean warming and a weakening land-sea thermal gradient There are large uncertainties looming over the status and fate of the South Asian summer monsoon, with several studies debating whether the monsoon is weakening or strengthening in a changing climate. Our analysis using multiple observed datasets demonstrates a significant weakening trend in summer rainfall during 1901–2012 over the central-east and northern regions of India, along the Ganges-Brahmaputra-Meghna basins and the Himalayan foothills, where agriculture is still largely rain-fed. Earlier studies have suggested an increase in moisture availability and land-sea thermal gradient in the tropics due to anthropogenic warming, favouring an increase in tropical rainfall. Here we show that the land-sea thermal gradient over South Asia has been decreasing, due to rapid warming in the Indian Ocean and a relatively subdued warming over the subcontinent. Using long-term observations and coupled model experiments, we provide compelling evidence that the enhanced Indian Ocean warming potentially weakens the land-sea thermal contrast, dampens the summer monsoon Hadley circulation, and thereby reduces the rainfall over parts of South Asia. The South Asian summer monsoon rainfall during June to September plays a significantly large role in the ‘roti and dal’ of roughly one-half of the world population [1] . The variability of the monsoon makes the region one of the most susceptible areas around the world to the impacts of climate-related natural disasters such as droughts and floods. Through observations and modelling, the scientific community has advanced its understanding of the past and future changes in the monsoons. With regard to the northern summer monsoon, some studies suggest that the monsoon circulation and rainfall have intensified in a changing climate [2] . Wang et al. [2] show that the rainfall over the northern hemisphere summer monsoon domain, as well as the Hadley and Walker circulations, have all undergone substantial intensification during the last three decades (1979–2011), with a striking increase of monsoon rainfall by 9.5% per degree of global warming. A few recent studies have also pointed out the increasing frequency of extreme rainfall events over the South Asian monsoon domain, due to a warming climate [3] . However, quite a few other studies indicate that the monsoon rainfall [4] , [5] , [6] and the Hadley and Walker circulations [7] , [8] , [9] are weakening over the South Asian domain during the past half century (since 1950s). Some of these studies suggest that, though the extreme rainfall events have increased over some regions [3] , the frequency of moderate-to-heavy rainfall events has decreased over the subcontinent [8] . In addition, several recent studies based on the Coupled Model Inter-comparison Project phase 5 (CMIP5) indicate a significant weakening of the large-scale Asian summer monsoon circulation, especially in the middle to upper atmosphere [10] , [11] , [12] . Monsoonal changes are found to be different when the region and time periods considered are different, and so are the implications [13] . In fact, a recent study [14] using proxy records for the Asian monsoon over the past two millennia suggests that the monsoon is currently in the decreasing phase of a multi-decadal oscillation. This study also cautions that monsoonal changes due to anthropogenic forcing will be difficult to detect against a backdrop of large natural variability. The Intergovernmental Panel on Climate Change (IPCC) Fifth Assessment Report (AR5) is also suggestive of the uncertainties looming over the status and fate of the monsoons [15] . Considering these uncertainties, there is an urgent need to provide robust information through the use of long-term observed datasets and climate models that could resolve the spatial and temporal lacuna associated with the monsoon variability in a changing climate. Climate models consistently show that, under increasing greenhouse gas forcing, the land-sea temperature contrast increases, possibly due to enhanced evaporation (latent heat loss) over the ocean [16] . An increase in the land-sea thermal contrast should ideally increase the strength of the monsoon [17] , [18] , [19] . Also, the sea surface temperatures (SST) over the Indian Ocean have shown a warming trend over the last several decades [20] , [21] , [22] , potentially enhancing the supply of moisture to the monsoon regions and increasing the rainfall amounts [23] . In a recent review of climate change and the South Asian monsoon, Turner and Annamalai [13] point out that though the land-sea contrast and the increased moisture availability should favour an increased monsoon rainfall, the observations do not provide any convincing evidence for such a positive trend. On the contrary, the South Asian monsoon rainfall has decreased significantly during the past several decades and this time evolution is not well reproduced by the CMIP5 models used in the IPCC AR5 (refs 4 , 11 , 12 , 24 , 25 , 26 ). This is indeed intriguing and escalates the uncertainty associated with the monsoon in a changing climate. In this study, we find that the summer monsoon rainfall during 1901–2012 shows a weakening trend over parts of South Asia. The reduction in rainfall is significant over the central-east and northern regions of India, along the Ganges-Brahmaputra basins and the Himalayan foothills (hereafter referred to as central Indian subcontinent), parts of India that are heavily populated and where agriculture is still mostly rain-fed. Using observations and climate model experiments, we demonstrate that this reduction in rainfall is linked to the rapid warming of the Indian Ocean, especially its western part, during the past century. The Indian Ocean warming, along with a relatively subdued warming of the Indian subcontinent, has played a key role in weakening the land-sea thermal contrast, a major driver of the South Asian monsoon. The weakened land-sea thermal contrast dampens the summer monsoon Hadley circulation, reducing the rainfall over the central Indian subcontinent. 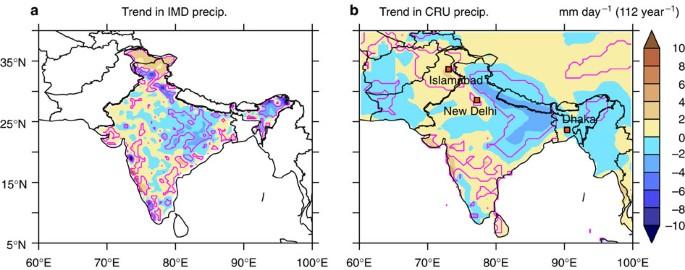Figure 1: Summer monsoon precipitation trends for the years 1901–2012. Observed trend in precipitation (mm day−1112 year−1) in (a) IMD and (b) CRU datasets, during June–September, for the years 1901–2012. Contours denote regions significant at the 95% confidence level. Rainfall trends during the past century Figure 1a,b shows the trend in precipitation over the South Asian region, during summer monsoon for the years 1901–2012, using gridded datasets from the India Meteorological Department (IMD) and the Climate Research Unit (CRU). The trends are similar in both the datasets, with a weakening trend over the central-east and northern regions of Indian subcontinent, and south of the Western Ghats region. The CRU dataset shows that the negative trend over the central subcontinent extends west to east, from south of Pakistan to central-east India, with a prominent horseshoe pattern with one of its arms placed on the foothills of the Himalayas, and the other obliquely along the central-east coast of India. The reduction in summer rainfall over central-east India during the past century is about 10–20%. This could have socio-economic consequences as the agriculture in this region is still largely rain-fed. Significant positive trends in precipitation are consistently observed to the north of the Western Ghats region, in both the datasets. However, the positive rainfall trends are confined to a small domain along the west coast. Figure 1: Summer monsoon precipitation trends for the years 1901–2012. Observed trend in precipitation (mm day −1 112 year −1 ) in ( a ) IMD and ( b ) CRU datasets, during June–September, for the years 1901–2012. Contours denote regions significant at the 95% confidence level. Full size image Warming Indian Ocean Previous studies using atmospheric general circulation models (AGCM) forced by observed SST variations suggest that a decrease in global land monsoon rainfall can be caused by warming trends over the tropical oceans, especially the central-eastern Pacific and the western Indian Ocean [27] . Among these tropical oceans, the Pacific SST anomalies do not show any long-term significant trend, while the western Indian Ocean exhibited rapid warming throughout the past century [28] ( Fig. 2 ). In comparison with the rest of the Indian Ocean, the western Indian Ocean generally has cooler mean SSTs in summer, owing to the strong monsoon winds and the resultant upwelling over the west. Meanwhile, the central-east Indian Ocean is characterized by a warm pool with SSTs greater than 28.0 °C. Though previous studies demonstrate a basin-wide warming in the Indian Ocean during the past half century [21] , [22] , our analysis using long-term SST datasets show that over an extended period of 112 years, the western Indian Ocean (WIO, 50–65°E, 5°S-10°N) has experienced anomalous warming of 1.2 °C ( Fig. 2 ), which is 0.5 °C greater than the warming over the warm pool region [28] . Even though a warming trend over the Indian Ocean may result in an increased supply of moisture locally over the ocean, it is not necessary that the surplus moisture is carried on to the peninsula [29] . The sustained Indian Ocean warming in the west has led to a greater westward extension of this Indian Ocean warm pool in recent decades [21] , [28] . The expansion of the Indian Ocean warm pool can in turn modify the land-sea thermal gradient, which could modulate the strength and flow of the monsoon circulation and the moisture laden winds towards the South Asian subcontinent. Hence, deciphering the relationship between the Indian Ocean warming and the monsoon precipitation might give a clue to the cause and effect of the observed rainfall trends over the region. 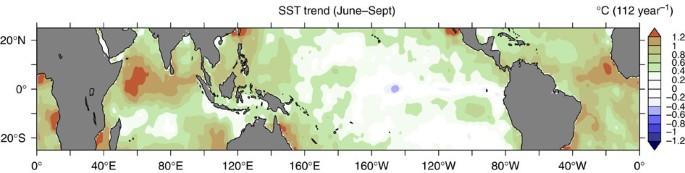Figure 2: Summer sea surface temperature trends for the years 1901–2012. Observed trend in mean summer (June–September) SST (°C 112 year−1) over the global tropics during 1901–2012. Figure 2: Summer sea surface temperature trends for the years 1901–2012. Observed trend in mean summer (June–September) SST (°C 112 year −1 ) over the global tropics during 1901–2012. Full size image To evaluate the association of the nearly monotonic warming over the western Indian Ocean on the observed monsoon trends over the subcontinent, we carried out a correlation analysis between SST and precipitation anomalies over the two regions. 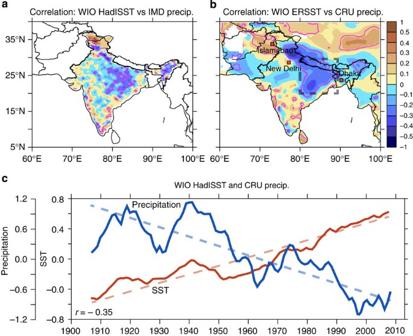Figure 3: Correlation between western Indian Ocean sea surface temperatures and monsoon precipitation. Correlation between SST over the western Indian Ocean (WIO, 50-65°E, 5°S-10°N) and precipitation over the South Asian subcontinent, for (a) HadISST and IMD precipitation, and (b) ERSST and CRU precipitation, for June–September 1901–2012. Contours denote regions significant at the 95% confidence level. The inset box includes parts of the central Indian subcontinent where the weakening trend in precipitation is significant (c) Time series of SST anomalies (°C,red) over western Indian Ocean along with CRU (blue) precipitation (mm day−1) over central Indian subcontinent (80–90°E, 20–30°N, inset box inb), smoothed with a 10 year moving average. Note that the correlation coefficient (r=−0.34) between HadISST and CRU precipitation is estimated using non-smoothed time series. Kendall’s rank correlation test for the two variables provided a tau coefficient of −0.3 (P<0.01, two tailed). Mann–Kendall test for the trend in the time series provided a tau coefficient of 0.6 for SST and −0.2 for precipitation, both significant at 95% confidence level. Figure 3a,b show the correlation between the western Indian Ocean SST anomalies and precipitation anomalies over the South Asian region, using multiple datasets. The spatial distribution of the correlation coefficients is consistent among the different data sets. The fascinating aspect is that, the correlation of precipitation anomalies with the Indian Ocean SST anomalies and the trend in these precipitation anomalies are strikingly similar. A pattern correlation computed between the trends in Fig. 1b and the correlation coefficients in Fig. 3b (for the region 60°–100°E, 5°–35°N at 0.5° horizontal grid resolution) indicates that they are strongly correlated ( r =0.73, significant at 95% confidence level). The most robust common feature among the trend and correlation patterns is a horseshoe pattern over central India. Apart from this, a dipolar pattern in the rainfall trends, with positive in the north and negative in the south is also visible along the Western Ghats of the Indian subcontinent ( Fig. 1 ). A recent study [30] suggests that enhanced warming to the north of western Indian Ocean in recent decades has also led to a poleward shift of the core of low-level monsoon winds, increasing the precipitation to the north of the Western Ghats, while weakening it over the south. This dipolar rainfall pattern between the south and north of the Western Ghats is also found to be associated with the western Indian Ocean warming at both the interannual and low frequency (for example, trend) timescales ( Fig. 3 ). Figure 3: Correlation between western Indian Ocean sea surface temperatures and monsoon precipitation. Correlation between SST over the western Indian Ocean (WIO, 50-65°E, 5°S-10°N) and precipitation over the South Asian subcontinent, for ( a ) HadISST and IMD precipitation, and ( b ) ERSST and CRU precipitation, for June–September 1901–2012. Contours denote regions significant at the 95% confidence level. The inset box includes parts of the central Indian subcontinent where the weakening trend in precipitation is significant ( c ) Time series of SST anomalies (°C, red ) over western Indian Ocean along with CRU ( blue ) precipitation (mm day −1 ) over central Indian subcontinent (80–90°E, 20–30°N, inset box in b ), smoothed with a 10 year moving average. Note that the correlation coefficient ( r =−0.34) between HadISST and CRU precipitation is estimated using non-smoothed time series. Kendall’s rank correlation test for the two variables provided a tau coefficient of −0.3 ( P <0.01, two tailed). Mann–Kendall test for the trend in the time series provided a tau coefficient of 0.6 for SST and −0.2 for precipitation, both significant at 95% confidence level. Full size image For a time series analysis, we consider the precipitation over the central Indian subcontinent (80–90°E, 20–30°N, inset box in Fig. 3b ) along with the western Indian Ocean SST anomalies ( Fig. 3c ). The rainfall region under consideration is chosen because the decreasing trend in rainfall is significant over this region, and also consistent with other studies utilizing station-wise analysis of rain gauge data [6] . Indeed, the SST and precipitation time series in Fig. 3c are negatively correlated ( r =−0.35 at df =110, for the unsmoothed time series), significant at 95% confidence level. Analysis using detrended time series data also shows significant negative correlation over the same region ( Supplementary Fig. 1 ). This means that similar processes may operate at interannual and lower frequency timescales to generate a secular downward monsoon rainfall trend in response to the warming of the western Indian Ocean, or alternatively, that a part of the Indian Ocean warming is due to the weakening of the monsoon [22] . The negative correlation is not observed during the first half of the 20th century, but becomes statistically significant post-1950s, probably due to the accelerated warming observed during the latter half. This implies that the relationship between a warm ocean and a weak monsoon is not linear. Since the ocean warming is a slow process, the heat has to build-up over several decades to make a substantial difference and reach the warm pool SST values (28.0 °C) [21] , [28] . The sustained western Indian Ocean warming has led to a greater spatial extension of the Indian Ocean warm pool in the recent decades only [21] . Changing land-sea thermal contrast As pointed out earlier, changes in the land-sea thermal contrast impact the strength of the monsoon [16] , [17] , [18] , [19] . Studies show that over the northern hemisphere, the surface temperatures over land increase more rapidly than over sea, under increasing greenhouse gases [19] . Ideally, such a scenario should strengthen the South Asian monsoon [16] , [17] , [18] , [19] . 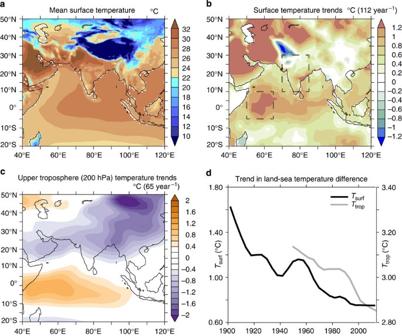Figure 4: Summer mean surface temperatures and land-sea temperature gradients for the years 1901–2012. Observed (a) mean (°C) and (b) trend (°C 112 year−1) of surface temperatures during June–September, 1901–2012. For the trend, the colour shades represent regions significant at the 95% confidence level. (c) Observed trend (°C 65 year−1) of upper tropospheric (200 hPa) temperatures during June–September, 1948–2012. (d) Time series of the trend in land-sea contrast in the surface (Tsurf) and tropospheric (Tsurf, 850-200hPa average) temperatures (°C). The land-sea contrast is estimated as the difference in the values between the boxes over the South Asian subcontinent (70–85°E, 10–30°N) and western Indian Ocean (50–65°E, 5°S-10°N), and the trend is estimated over 31 year sliding periods. The land surface temperature is from HadCRUT, SST from HadISST and tropospheric temperature from NCEP reanalysis. Figure 4a,b shows the climatological mean and trends of surface temperatures over the Indian Ocean and the South Asian monsoon domain, during summer. Obviously, the monotonic warming trend over the Indian Ocean is prominent, with the strongest warming over the west. At the same time the Indian subcontinent exhibits suppressed warming during the past century. In fact, the surface temperatures in the northern Indian peninsula show a cooling trend. This implies a weakening meridional thermal gradient over the South Asian domain, in contrast with earlier studies that suggest a strengthening of the thermal gradient under a globally warming scenario. The weakening land-sea thermal gradient is reproduced in other datasets also, indicating the robustness of the trend ( Supplementary Fig. 2 ). Figure 4: Summer mean surface temperatures and land-sea temperature gradients for the years 1901–2012. Observed ( a ) mean (°C) and ( b ) trend (°C 112 year −1 ) of surface temperatures during June–September, 1901–2012. For the trend, the colour shades represent regions significant at the 95% confidence level. ( c ) Observed trend (°C 65 year −1 ) of upper tropospheric (200 hPa) temperatures during June–September, 1948–2012. ( d ) Time series of the trend in land-sea contrast in the surface ( T surf ) and tropospheric ( T surf , 850-200hPa average) temperatures (°C). The land-sea contrast is estimated as the difference in the values between the boxes over the South Asian subcontinent (70–85°E, 10–30°N) and western Indian Ocean (50–65°E, 5°S-10°N), and the trend is estimated over 31 year sliding periods. The land surface temperature is from HadCRUT, SST from HadISST and tropospheric temperature from NCEP reanalysis. Full size image The land-sea contrast in surface temperatures, though important, may not provide a comprehensive picture of the factors modulating the strength of the monsoon circulation. Once the monsoon rains set in on the South Asian subcontinent, the land surface cools down considerably. However, the troposphere above the land remains warm due to the latent heat release from the convective activity, keeping the thermal contrast functional [31] . This means that the tropospheric temperature is an ideal parameter for examining the thermodynamic forcing related to the monsoon [31] . However, unlike the surface temperature, robust records of air temperature at different levels of the troposphere are not available before the 1950s, which makes it difficult to examine the role of long-term tropospheric temperature trends on the monsoon. Nevertheless, to confirm that our results are valid for the recent decades also, we analyse the tropospheric temperatures over the monsoon domain. The trend in the thermal contrast is well reflected in the upper tropospheric (200 hPa) temperature anomalies also, as demonstrated in Fig. 4c . Along with a cooling trend over the larger Indo-Tibetan landmass, increasing positive temperature anomalies are observed over the western Indian Ocean, indicating its potential role in weakening the monsoon flow towards the Indian peninsula. The warming of the upper troposphere over the Indian Ocean ( Fig. 4c ) is co-located with that over the sea surface ( Fig. 4b ). This may be attributed to the fact that the tropical Indian Ocean is a highly convective region during the northern summer, as the mean SSTs are above the minimum convective threshold (26 °C) and the southwesterly monsoon winds are conducive for enhanced moisture convergence [32] . Further warming of the Indian Ocean enhances the convection [23] , transferring surplus heat to the upper troposphere [33] , [34] , [35] . To evaluate the trends observed in land-sea thermal contrast in Fig. 4b,c , we analyse the difference between the summer tropospheric temperatures over western Indian Ocean and the Indian subcontinent, at 850 and 200 hPa levels ( Fig. 4d ). The surface temperature gradient ( T surf ) shows a sharp decline throughout the past century, largely contributed by an increased warming over the western Indian Ocean. The tropospheric temperature gradient ( T trop ) post-1950s also indicates a trend similar to that in the surface temperatures. This is suggestive of a warm Indian Ocean having a strong hold on the whole troposphere, from the surface to the top, possibly due to enhanced convective mixing over the ocean [33] , [34] , [35] . Indeed, a separate analysis of the trend at each of these levels gave consistent results of a warming troposphere over the Indian Ocean, and a weakening thermal contrast between the subcontinent and the ocean. All these results indicate a reduced land-sea thermal contrast during the past century, partly due to increased warming over the Indian Ocean, especially over the western region, and partly due to a relatively weaker warming over the Indian peninsula. Weakening of the summer monsoon Hadley circulation Many studies have shown that warm SST anomalies are accompanied by large variations in the lower and upper troposphere due to enhanced latent heating aloft from convection over the ocean [33] , [34] , [35] . Furthermore, these changes are highly correlated with the strength of the monsoon circulation [31] , [34] . A more recent study using a coupled model framework also points out that a spatial extension of Indian Ocean warm pool could enhance the convection over the ocean while introducing a dry bias over land, by modulating the meridional Hadley circulation [36] . It is therefore likely that the impact of the Indian Ocean warming on the monsoon has become more prominent in recent decades. Consistently, an examination of the vertical wind velocity over the South Asian domain (50–100°E) during the years 1948–2012 indicates largescale upward motion over the equatorial ocean (10°S-10°N), extending up to the upper troposphere and favouring intense local convection ( Fig. 5a ). Furthermore, this enhanced upward motion over the ocean is compensated by subsidence of air over the subcontinent (10–20°N), inhibiting convection over the landmass and drying the region, through a modulation of the local Hadley cell ( Fig. 5a ). This suggests that though the warming ocean engenders enhanced local rainfall due to increased moisture availability, it weakens the monsoon Hadley circulation and reduces the rainfall over the land, ultimately building up a competition among the land and ocean rainfall in the South Asian monsoon domain. 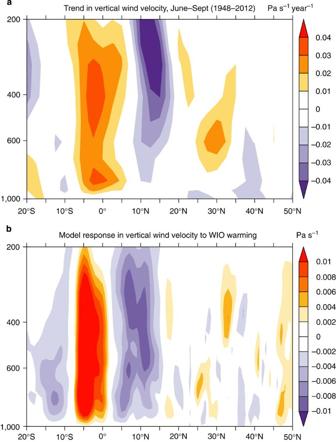Figure 5: Observed trends and model simulated changes in summer monsoon Hadley circulation in response to Indian Ocean warming. (a) Trend from NCEP re-analysis (Pa s−1year−1) and (b) model simulated response (Pa s−1) to western Indian Ocean warming in vertical velocity (omega) during northern summer (June–September) along the South Asian domain (50–100°E). Positive (red) values indicate upward motion. Figure 5: Observed trends and model simulated changes in summer monsoon Hadley circulation in response to Indian Ocean warming. ( a ) Trend from NCEP re-analysis (Pa s −1 year −1 ) and ( b ) model simulated response (Pa s −1 ) to western Indian Ocean warming in vertical velocity (omega) during northern summer (June–September) along the South Asian domain (50–100°E). Positive (red) values indicate upward motion. Full size image Climate model response to Indian Ocean warming Attribution of the decreasing monsoon rainfall to the Indian Ocean warming from observations alone is very difficult and probably impossible. Thus, to delineate and examine the role of the Indian Ocean warming on the monsoon circulation and rainfall, model sensitivity experiments using an ocean-atmosphere coupled climate model were carried out. In the sensitivity experiment, positive SST anomalies similar to those in the observations were added to the western Indian Ocean region ( Supplementary Fig. 3 ). Figure 5b shows the model response in the summer monsoon Hadley circulation, and features a weakening of the local Hadley cell, much similar to the observed trends. The fact that the warming has resulted in enhanced convection over the ocean and subsidence over the landmass serves as the evidence that the observed warming trend in the Indian Ocean has the potential to weaken the monsoon circulation. 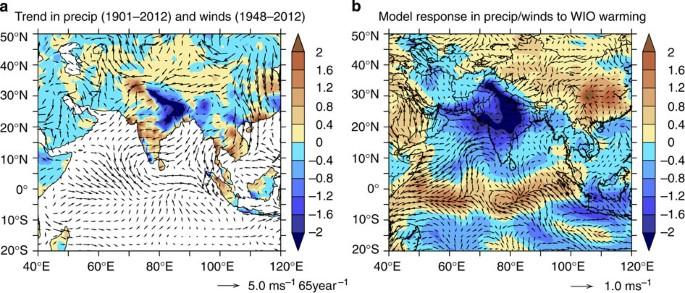Figure 6: Observed trends and model simulated changes in summer monsoon precipitation in response to Indian Ocean warming. (a) Observed trend in precipitation (CRU data, 1901–2012, mm day−1) and near-surface winds (NCEP, 1948–2012, m s−1), for June-September. (b) Model-simulated mean precipitation (mm day−1) and wind (10 m) anomalies (m s−1) in response to warming over the western Indian Ocean. The model-simulated anomalies are estimated from the sensitivity run where SST anomalies of the order of 1.5 °C is introduced over the western Indian Ocean (CFSv2WIO), with respect to a model control run (CFSv2CTL). Figure 6 compares the observed trends in precipitation and surface winds with the model-simulated anomalies in response to warming over the western Indian Ocean. The interesting, robust element in the model simulations ( Fig. 6b ) is the horseshoe pattern in the negative precipitation anomalies, with one arm placed over the Himalayan foothills and the other over the central Indian landmass, similar to the one in the precipitation trends ( Figs 1 and 6a ) and the correlation pattern with western Indian Ocean SST anomalies ( Fig. 3a,b ). Consistent with the reduced precipitation, the surface winds also suggest weakened mean southwesterly winds. The trend analysis ( Fig. 6a ) shows a Rossby wave-like response [37] to the Indian Ocean warming, with northeasterly wind anomalies over most of the Arabian Sea, converging towards the central Indian Ocean. The model simulation ( Fig. 6b ) also shows similar results, with respect to the Rossby wave response near the subcontinent and over the Arabian Sea. However, the zonal direction of the wind anomalies near the equator appears different in the observations and the model. This is not an unexpected result as the periods under consideration and the model simulations are different, since the observed winds are available only for 1948–2012, a period during which the Indian Ocean experienced a basin-wide warming [21] , [22] . In fact previous studies using AGCM experiments driven by recent basin-wide warming in the tropical Indian Ocean reproduced the observed zonal wind changes in the recent decades [38] . In the model sensitivity experiment, however, the positive SST offset is prescribed only over the western Indian Ocean region, where the long-term warming trend is observed in the SST records during 1901–2012. This suggests that while western Indian Ocean warming plays a significant role in the long-term change in winds, basin-wide warming over the tropical Indian Ocean has emerged as a co-conspirator in the change in land-sea thermal contrast and winds in recent decades. Figure 6: Observed trends and model simulated changes in summer monsoon precipitation in response to Indian Ocean warming. ( a ) Observed trend in precipitation (CRU data, 1901–2012, mm day −1 ) and near-surface winds (NCEP, 1948–2012, m s −1 ), for June-September. ( b ) Model-simulated mean precipitation (mm day −1 ) and wind (10 m) anomalies (m s −1 ) in response to warming over the western Indian Ocean. The model-simulated anomalies are estimated from the sensitivity run where SST anomalies of the order of 1.5 °C is introduced over the western Indian Ocean (CFSv2 WIO ), with respect to a model control run (CFSv2 CTL ). Full size image A further comparison of the model response to the warming is provided in Supplementary Fig. 4 . The thermal response (surface and upper troposphere) is similar to those in the observed trends over the ocean, but exhibit some discrepancies over land. More specifically, for the model response in temperature at 200 hPa, the results reproduce the upper tropospheric warming over the ocean, but do not replicate the cooling over the Indo-Tibetan landmass. This is possibly because of the role of other processes on the upper tropospheric temperatures, such as aerosol forcing [39] , [40] and stratosphere–troposphere interactions [41] , which are not included in the model experiment. It may also be noted that previous studies [41] have suggested that the NCEP upper tropospheric data overestimate the cooling trend over the Indo-Tibetan landmass. Nevertheless, the similarity between the rainfall and local Hadley responses between the model experiments and observed fields clearly demonstrates the importance of western Indian Ocean warming in determining the observed monsoon response. The above analysis using observations and climate model sensitivity experiments indicates the potential role of the Indian Ocean warming in weakening the monsoon circulation and rainfall over central Indian subcontinent. The Indian Ocean and monsoon exhibit a coupled relationship [32] , [42] , [43] , and it is also possible that a feedback from a weak monsoon accelerates the warming in the Indian Ocean [22] . Some studies have suggested a role for anthropogenic aerosols in weakening the monsoon circulation during the recent decades [40] , [44] , [45] , [46] , [47] , [48] . It is possible that such a weakened circulation amplifies the SST warming due to a decreased evaporation. In contrast, recent studies show that the anthropogenic aerosols tend to have a cooling effect and compete with the greenhouse warming over the Indian Ocean [49] , [50] . Despite the fact that aerosols are a competing factor, the observed SST trends do not show any change during the post-1980s where aerosols have increased ( Fig. 3c ). In fact, a study [50] points out that a large share of the CMIP5 models with aerosol forcing is not able to reproduce the observed SST warming over the Indian Ocean. They attribute this issue to the large uncertainties in representing the direct and indirect effects of aerosols in these models. Meanwhile, a recent study demonstrates that apart from the warming due to greenhouse gas forcing [51] , the long-term warming trend in the western Indian Ocean is significantly associated with the asymmetry in the ENSO forcing [28] . That is, while the quasi-periodic El Niño events induce a warming over the Indian Ocean via the Walker circulation, the La Niña events fail to do the inverse. Along with this, an increase in the magnitude and frequency of El Niños in the recent decades has accelerated this warming [28] . The heat pile-up due to this ENSO forcing [52] persists in the land-locked Indian Ocean that has a restricted thermohaline circulation, sustained by a feedback from the local air-sea interaction [53] , [54] and ocean dynamics [55] , [56] . Considering the strong seasonal variability in this region and short-term persistence in atmospheric changes, it is rather self-evident that, on longer time scales, the warmer ocean plays a larger role in weakening the monsoon than vice-versa. Though the observed increase in anthropogenic aerosols may not have a direct effect in warming the Indian Ocean, they may have a potential role in suppressing (or even cooling) the surface warming over the South Asian domain in the recent decades [39] , [40] . Aerosols could be considered as the perfect partner in reducing the land-sea thermal contrast, along with a warming Indian Ocean. An evaluation of the CMIP5 models [40] suggests that aerosols could potentially reduce the incoming solar radiation over the Indo-Gangetic plain, thereby cooling the surface. However, it may be pointed out that majority of these models could not simulate the spatial distribution of aerosols or related processes over the South Asian subcontinent [40] . Also, ambiguity still remains on the extent of cooling (or warming) induced by different types of aerosols [45] , [46] , [47] . Meanwhile, other studies link the upper tropospheric cooling over the larger Indo-Tibetan landmass during summer to stratospheric temperature changes that are channelled through stratosphere–troposphere interactions [41] . Further research is required to differentiate the individual contributions of these components on the observed trends in surface and upper tropospheric temperatures over land. The current study discusses the role of Indian Ocean warming in weakening of the monsoon, but does not rule out the possibility that similar impacts may also arise due to SST changes in the tropical Pacific and the Atlantic [9] , [54] , [57] , [58] , [59] , [60] , [61] . Recent studies show that the Pacific warming trend during the past century is not prominent as compared with the Indian Ocean warming while the tropical and extratropical Atlantic show strong warming trends [28] . However, Prodhomme et al. [61] pointed out that a warming in the tropical Atlantic does not change the tropospheric temperature gradient between the Indian Ocean and the subcontinent as the temperature changes due to the teleconnection are uniform over this domain. Meanwhile, Goswami et al. [59] suggest that a North Atlantic warming should ideally strengthen the Asian monsoon by increasing the tropospheric temperatures over northern India and southern Eurasia. However, temperature and rainfall trends during recent decades suggest that any such role of the Atlantic is offset by the tropospheric temperature trends induced by a warming Indian Ocean. Deconvolving the non-stationary relations between the monsoon and the warming over these remote regions is beyond the scope of this study. But considering the robustness of the Indian Ocean warming and its direct role in monsoon dynamics in comparison with the other tropical oceans, it is justified to say that the Indian Ocean SST trends play a relatively larger role on the observed rainfall trends in the South Asian domain. A recent study comparing present observations and future regional climate model projections of the summer monsoon suggests a further weakening of the monsoon circulation and peninsular rainfall in the future [62] . Meanwhile, the CMIP5 future projections suggest an increase in rainfall over the central Indian subcontinent [26] , though one must note the ongoing debate about whether CMIP5 models are in fact capturing the historic monsoon trends accurately [4] , [11] , [12] , [24] and whether the monsoon projections are reliable in these models [25] . The overall weakening trend of monsoon rainfall over South Asia is a matter of grave concern since the socio-economic livelihood in this region, including agriculture, water resources and power generation are irrevocably dependent on it. The role of Indian Ocean warming might not be solely limited to weakening the Asian monsoon. Research based on climate proxy records and models point out that the climate signals forced by warm SST anomalies over the tropical Indian and western Pacific oceans synergistically contribute to widespread drying over South Asia and mid-latitudes, an ideal scenario for a large-scale drought [63] , [64] . In addition, a recent study points out that the Indian Ocean warming may also be playing an important role in modulating the Pacific climate change in recent decades, by favouring stronger trade winds in the Pacific, thereby contributing to the recent global warming hiatus [65] . Hence, the critical role of the warm Indian Ocean deserves special attention not only for its decisive effect on the food security of a large fraction of the world’s population, but also due to its disproportionately large role as a partner to the warm pool Pacific in inducing a drought, as well as its potential role in the global warming pause. Rainfall and SST historical data analysis Two long-term precipitation datasets for the northern summer during the period 1901–2012, obtained from the India Meteorological Department (IMD) and Climate Research Unit (CRU) are used in this study. The recent IMD precipitation data use daily rainfall data from all the rain gauge stations over India, gridded at 0.25° horizontal resolution [66] . This includes rainfall records from 6,955 stations, which is the highest number of stations used by any gridded datasets currently available. The data density varies from year to year from about 1,500 in the first couple of years to about 4,000 by the end of the century. The trend in precipitation over the central Indian region under consideration is compared with studies utilizing station wise analysis of rain gauge data [6] . SST data for the same period are obtained from the HadISST1 dataset provided by the Met Office Hadley Centre, and also the Extended Reconstructed Sea Surface Temperature (ERSST) provided by NOAA. To examine the role of land-sea temperature gradient, surface temperatures from HadCRUT (1901–2012) and tropospheric temperature values from NCEP reanalysis (1948–2012) are used. Observed trends in the monsoon southwesterlies are inferred from the wind data based on NCEP reanalysis during 1948–2012. The significance of the trends and correlations is examined using standard two-tailed Student’s t -tests. The correlation analysis in Fig. 3c has also been tested using Kendall’s rank correlation that is non-parametric and therefore makes no assumptions about the distribution and at the same time determine the direction and significance of the relation between the two variables [67] . The correlated variables are said to be concordant if their ranks vary together (−1) and discordant if they vary differently (+1). The significance of the rainfall and SST linear trend values are further assessed with Mann–Kendall tests [68] with block bootstrap to improve the significance test when a time series shows auto-correlation. Model and experimental design For the numerical model experiments, we use the standard configuration of a global coupled ocean-atmosphere model, the Climate Forecast System version 2 (CFSv2). The CFSv2 model simulates the mean monsoon and its interannual variability reasonably well, and hence used in this study [42] . The oceanic component has a 0.25–0.5° horizontal resolution, 40 vertical levels and includes an ice model. The atmospheric component is at T126 ( ∼ 0.9°) horizontal resolution and 64 sigma-pressure hybrid levels. The atmosphere and ocean exchange quantities such as heat and momentum fluxes every half an hour, with no flux adjustment or correction. See Saha et al. [69] for further details on the model and its components. The coupled configuration of CFSv2 is time integrated over a period of 100 years, and utilized as the reference run (CFSv2 CTL ). To examine the role of a warming Indian Ocean, a sensitivity experiment (CFSv2 WIO ) using ensembles (20 members) of short integrations for the summer monsoon season during June–September were performed by adding temperature anomalies to the SSTs passed over the western Indian Ocean, to the atmosphere. Positive anomalies of the order of 1.5 °C were added over the region, in such a way that it tapers out by the limits of the domain (50–65°E, 5°S–10°N). The positive offset added to the simulated SSTs over western Indian Ocean in the sensitivity experiments is similar to the amplitude of the observed trends ( Fig. 2 , Supplementary Fig. 3 ). The difference between CFSv2 WIO and CFSv2 CTL is taken as the model response to the summer warming over the western Indian Ocean. Accession codes: The climate model code utilized in this study, the NCEP Climate Forecast System version 2, is available at the ‘Monsoon Desk’ at NOAA’s National Centres for Environmental Prediction (NCEP), as part of the National Monsoon Mission setup by the Ministry of Earth Sciences, Government of India [url: http://www.emc.ncep.noaa.gov/index.php?branch=monsoondesk ]. How to cite this article: Roxy, M. K. et al. Drying of Indian subcontinent by rapid Indian Ocean warming and a weakening land-sea thermal gradient. Nat. Commun. 6:7423 doi: 10.1038/ncomms8423 (2015).